Nuclear receptor NR4A1 promotes breast cancer invasion and metastasis by activating TGF-β signalling In advanced cancers, the TGF-β pathway acts as an oncogenic factor and is considered to be a therapeutic target. Here using a genome-wide cDNA screen, we identify nuclear receptor NR4A1 as a strong activator of TGF-β signalling. NR4A1 promotes TGF-β/SMAD signalling by facilitating AXIN2–RNF12/ARKADIA-induced SMAD7 degradation. NR4A1 interacts with SMAD7 and AXIN2, and potently and directly induces AXIN2 expression. Whereas loss of NR4A1 inhibits TGF-β-induced epithelial-to-mesenchymal transition and metastasis, slight NR4A1 ectopic expression stimulates metastasis in a TGF-β-dependent manner. Importantly, inflammatory cytokines potently induce NR4A1 expression, and potentiate TGF-β-mediated breast cancer cell migration, invasion and metastasis in vitro and in vivo . Notably, NR4A1 expression is elevated in breast cancer patients with high immune infiltration and its expression weakly correlates with phosphorylated SMAD2 levels, and is an indicator of poor prognosis. Our results uncover inflammation-induced NR4A1 as an important determinant for hyperactivation of pro-oncogenic TGF-β signalling in breast cancer. Transforming growth factor (TGF)-β signalling plays critical roles in embryonic development and the maintenance of tissue homoeostasis in all metazoans [1] , [2] , [3] . TGF-β signals via specific complexes of type I and type II Ser/Thr kinase receptors. The activated TGF-β type I receptor (TβRI) induces SMAD2/3 phosphorylation; phosphorylated SMAD2/3 forms hetero-oligomers with SMAD4, which accumulate in the nucleus to regulate the expression of target genes [4] , [5] . SMAD7 functions as an inhibitory SMAD by recruiting the E3 ligase SMURF1/2 to the type I receptor and subsequently degrading TβRI and mitigating TGF-β signalling [6] , [7] . ARKADIA and RNF12 potentiate TGF-β signalling by targeting SMAD7 for polyubiquitination and degradation [8] , [9] . Deregulation of TGF-β activity can result in cancer development. In normal and premalignant cells, TGF-β enforces homoeostasis and suppresses tumour progression directly through cell autonomous regulation of apoptosis and growth arrest or indirectly through blockage of paracrine factor production in the tumour stroma. However, when cancer cells lose the TGF-β tumour suppressive responses, they can utilize TGF-β as a potent promoter of cell motility, invasion, metastasis and tumour stem cell maintenance [1] , [10] . NR4A1 (also named Nur77, TR3 or NGF-IB) is a member of the steroid/thyroid hormone receptor superfamily. It is a transcription factor and as an early response gene, it can be induced by many stimuli including serum, inflammatory factors, growth factors and stress in different cell types and organs [11] . NR4A1 was considered as a strong tumour suppressor because of its involvement in growth inhibition and induction of apoptosis [12] , [13] , [14] , [15] . Nevertheless, NR4A1 was also reported to be highly expressed in colon and pancreatic tumours. Knockdown of NR4A1 in these cancer cells resulted in inhibition of cell growth, induction of apoptosis and decreased angiogenesis [16] , [17] . These findings suggest that NR4A1 has both a tumour suppressive and pro-oncogenic effect in cancer development. In this study, we discovered NR4A1 expression as a highly potent TGF-β/SMAD signalling activator by inducing the degradation of SMAD7. Moreover, we demonstrate that inflammation-induced NR4A1 greatly potentiates TGF-β-induced breast cancer cell invasion and metastasis. NR4A1 is an activator of TGF-β/SMAD signalling To identify novel regulators of TGF-β signalling, a genome-wide gene-by-gene screen was conducted. The Origene10K (two sets) and MGC7K complementary DNA libraries [18] (total 27,000 genes) were screened in duplicate in HEK293T cells stably transfected with the SMAD3/SMAD4-dependent CAGAR 12 -Luc transcriptional reporter stimulated with a suboptimal dose of TGF-β. Among the screened cDNAs, nuclear receptor NR4A1 was identified as one of the top three activators of TGF-β/SMAD signalling ( Fig. 1a and Supplementary Fig. 1 ). Consistently, in a short interfering RNA screen depleting 5,000 druggable genes one by one in the same reporter cell line, siNR4A1 was identified as an inhibitor of this response ( Fig. 1b ). NR4A1 promoted TGF-β/SMAD transcription to a greater extent compared with SMAD3, whereas short hairpin RNA (shRNA)-mediated NR4A1 depletion decreased TGF-β/SMAD transcription ( Fig. 1c ). 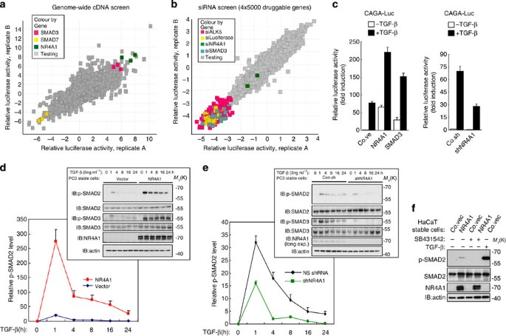Figure 1: NR4A1 is screened as an activator of TGF-β/SMAD signalling. (a) A genome-wide cDNA overexpression screen in HEK 293T cells using TGF-β-induced CAGA12-luc transcriptional response as assay. Three NR4A1 cDNAs that potently stimulated the luciferase activity were identified. As expected, SMAD3 and SMAD7 stimulated and inhibited the luciferase activity, respectively. (b) Short interfering RNA (siRNA) screening chart for 5,000 druggable genes in which two NR4A1 siRNA were identified that repressed the luciferase activity. siALK5, siLuciferase and siSMAD3 that strongly repress luciferase activity served as positive controls. The x and y axes are the relative luciferase activity in two replicates inaandb. (c) Validation of NR4A1 overexpression or knockdown for SMAD3 transcriptional response induced by TGF-β (5 ng ml−1) in HEK293T cells. Data are presented as mean±s.d. (n=3 measurements). NS shRNA, non-targeting shRNA; RLU, relative luciferase units. (d) Immunoblot (IB) analysis of PC3 cells stably expressing NR4A1. (e) Immunoblot (IB) analysis of PC3 cells stably depleted of NR4A1 by shRNA (shNR4A1). (f) HaCaT cells stably expressing NR4A1 were treated with TGF-β (1 ng ml−1) or SB431542 (10 μM) for 1 h and then lysed for immunoblot analysis. Figure 1: NR4A1 is screened as an activator of TGF-β/SMAD signalling. ( a ) A genome-wide cDNA overexpression screen in HEK 293T cells using TGF-β-induced CAGA12-luc transcriptional response as assay. Three NR4A1 cDNAs that potently stimulated the luciferase activity were identified. As expected, SMAD3 and SMAD7 stimulated and inhibited the luciferase activity, respectively. ( b ) Short interfering RNA (siRNA) screening chart for 5,000 druggable genes in which two NR4A1 siRNA were identified that repressed the luciferase activity. siALK5, siLuciferase and siSMAD3 that strongly repress luciferase activity served as positive controls. The x and y axes are the relative luciferase activity in two replicates in a and b . ( c ) Validation of NR4A1 overexpression or knockdown for SMAD3 transcriptional response induced by TGF-β (5 ng ml −1 ) in HEK293T cells. Data are presented as mean±s.d. ( n =3 measurements). NS shRNA, non-targeting shRNA; RLU, relative luciferase units. ( d ) Immunoblot (IB) analysis of PC3 cells stably expressing NR4A1. ( e ) Immunoblot (IB) analysis of PC3 cells stably depleted of NR4A1 by shRNA (shNR4A1). ( f ) HaCaT cells stably expressing NR4A1 were treated with TGF-β (1 ng ml −1 ) or SB431542 (10 μM) for 1 h and then lysed for immunoblot analysis. Full size image Stably expressing NR4A1 in PC3 prostate cancer cells highly potentiated TGF-β-induced SMAD2 and SMAD3 phosphorylation, whereas PC3 cells with stable NR4A1 knockdown dramatically decreased these responses ( Fig. 1d,e ). Ectopic NR4A1 expression increased SMAD2/3–SMAD4 complex formation, even without TGF-β stimulation, whereas shRNA-mediated NR4A1 depletion reduced complex formation ( Supplementary Fig. 2a,b ). SMAD2/3 nuclear translocation was enhanced by NR4A1 expression and diminished by NR4A1 depletion ( Supplementary Fig. 2c ). In addition, when ectopically expressed in HaCaT cells, NR4A1 promoted SMAD2 phosphorylation, even without the addition of TGF-β ligand. This result was due to autocrine TβRI activation because the TβRI kinase inhibitor compound (SB431542) blocked this induction ( Fig. 1f ). Moreover, subcutaneous injection of head and neck cancer, head and neck (HN)5 cells expressing NR4A1 led to the high SMAD3 transcriptional HN5 cell autonomous activity in vivo mediated by endogenous TGF-β-like ligands without significant difference in cell proliferation ( Fig. 2a–c , Supplementary Fig. 3a,b and data not shown). Furthermore, phospho-SMAD2 was greatly induced in mouse livers infected with adenovirus expressing NR4A1, indicating in situ activation of the TGF-β signal by NR4A1 ( Fig. 2d,e and Supplementary Fig. 3c ). Compared with wild-type mouse embryonic fibroblasts (MEFs), TGF-β-induced phospho-SMAD2 was decreased in primary NR4A1 −/− MEFs ( Fig. 2f ). Consistent with this finding, two direct target genes of TGF-β/SMAD, that is, SMAD7, which participates in a negative feedback loop and connective tissue growth factor ( CTGF) , were downregulated in NR4A1 −/− MEF cells compared with wild-type MEFs ( Fig. 2g ). In addition, in breast cancer patients, we observed strong and significant positive correlation between NR4A1 and TGF-β/SMAD direct target genes PAI-1 (plasminogen activator inhibitor-1)/ CTGF , as well as weak but also significant correlation between NR4A1 and Smad7/CXCR4 ( CXC chemokine receptor 4; Fig. 2h ). Thus, NR4A1 greatly activates and is a strong and important, but not essential, determinant of TGF-β/SMAD signalling. 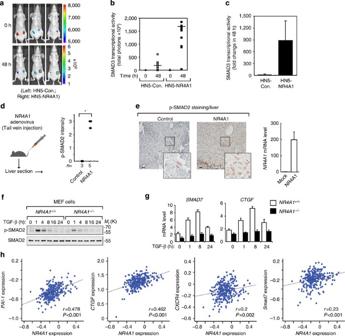Figure 2: NR4A1 drives TGF-β/SMAD signallingin vivoand is critically required for TGF-β/SMAD activation. (a–c)In vivoSMAD3 transcriptional activity analysis. (a) Bioluminescent imaging of three representative mice at 0 and 48 h injected with HN5-luc cells stably expressing green fluorescence protein control (left-hand-side xenograft ) and NR4A1 (right-hand-side xenograft). (b) SMAD3 transcriptional activity from 0 to 48 h presented in total photons. Data are presented as mean±s.d. (n=8). (c) The average and s.d. of fold change of left pannel. (d) Tail vein injection of adenovirus expressing NR4A1 led to elevated levels of phospho-SMAD2 in the mouse liver. The intensity of phospho-SMAD2 staining is analysed. For mock,n=3; for NR4A1,n=5. (*P<0.05 by Student’st-test). (e) Representative images of p-SMAD2 immunohistochemistry results are shown. Left panel, representative immunohistochemical (IHC) staining of phospho-SMAD2 in mouse livers. Red arrow indicates representative nuclear phospho-SMAD2 signal. Scale bar, 70 μm. Right panel, qRT–PCR identification of NR4A1 expression in mouse liver. Data are presented as mean±s.d. (n=3). (f) IB analysis ofNR4A1+/+andNR4A1−/−primary MEFs treated with TGF-β (5 ng ml−1) for the indicated time. (g) qRT–PCR analysis of TGF-β target genes inNR4A1+/+andNR4A1−/−MEFs treated with TGF-β (5 ng ml−1) for the indicated times. Data are presented as mean±s.d. (n=3). (h) Scatter plot showing the positive correlation betweenNR4A1andSMAD7/PAI-1/CTGF/CXCR4expression in the NKI295 clinical data set (n=295). Pearson’s’ coefficient tests were performed to assess statistical significance. Figure 2: NR4A1 drives TGF-β/SMAD signalling in vivo and is critically required for TGF-β/SMAD activation. ( a – c ) In vivo SMAD3 transcriptional activity analysis. ( a ) Bioluminescent imaging of three representative mice at 0 and 48 h injected with HN5-luc cells stably expressing green fluorescence protein control (left-hand-side xenograft ) and NR4A1 (right-hand-side xenograft). ( b ) SMAD3 transcriptional activity from 0 to 48 h presented in total photons. Data are presented as mean±s.d. ( n =8). ( c ) The average and s.d. of fold change of left pannel. ( d ) Tail vein injection of adenovirus expressing NR4A1 led to elevated levels of phospho-SMAD2 in the mouse liver. The intensity of phospho-SMAD2 staining is analysed. For mock, n =3; for NR4A1, n =5. (* P <0.05 by Student’s t -test). ( e ) Representative images of p-SMAD2 immunohistochemistry results are shown. Left panel, representative immunohistochemical (IHC) staining of phospho-SMAD2 in mouse livers. Red arrow indicates representative nuclear phospho-SMAD2 signal. Scale bar, 70 μm. Right panel, qRT–PCR identification of NR4A1 expression in mouse liver. Data are presented as mean±s.d. ( n =3). ( f ) IB analysis of NR4A1 +/+ and NR4A1 −/− primary MEFs treated with TGF-β (5 ng ml −1 ) for the indicated time. ( g ) qRT–PCR analysis of TGF-β target genes in NR4A1 +/+ and NR4A1 −/− MEFs treated with TGF-β (5 ng ml −1 ) for the indicated times. Data are presented as mean±s.d. ( n =3). ( h ) Scatter plot showing the positive correlation between NR4A1 and SMAD7 / PAI-1 / CTGF / CXCR4 expression in the NKI295 clinical data set ( n =295). Pearson’s’ coefficient tests were performed to assess statistical significance. Full size image NR4A1 accelerates SMAD7 degradation Enhancement of phospho-SMAD2 by NR4A1 suggests NR4A1 acts upstream of SMAD2/3. In addition, we found that NR4A1 did not induce SMAD3, SMAD4 and ALK5 expression at the messenger RNA level. Thus, NR4A1 does not appear to cooperate with SMAD3 as a transcription factor, nor does it induce the expression of agonistic TGF-β receptor/SMAD signalling mediators, to facilitate TGF-β/SMAD signalling. We next tested whether NR4A1 misexpression affects TβRI levels at the plasma membrane, where signalling is initiated [19] . Upon ectopic expression with NR4A1, biotin-labelled cell surface TβRI displayed a prolonged half-life ( Fig. 3a ). In line with this, NR4A1 depletion in MDA-MB-231 cells led to lower cell surface TβRI levels and accelerated degradation ( Fig. 3b ). SMAD7 functions as an inhibitory SMAD by recruiting E3 ligase SMURF1/2 to the type I receptor and subsequently degrading TβRI and mitigating TGF-β signalling [6] , [7] . Indeed, in NR4A1 stably depleted PC3 cells, we found that the polyubiquitination of TβRI was increased ( Supplementary Fig. 4a ). Interestingly, NR4A1 did not bind to R-SMAD and SMAD4, but specifically bound inhibitory SMAD7 ( Fig. 3c ). This made us analyse the effect of NR4A1 on SMAD7 protein expression. SMAD7 protein (in contrast to SMAD7 mRNA) was downregulated in PC3 cells stably expressing NR4A1 ( Fig. 3d ). Conversely, in NR4A1 stably depleted cells, SMAD7 was upregulated. Consistent with this, we observed that TβRI inversely correlated with SMAD7 level, and was upregulated and downregulated in NR4A1 stably expressing and depleted cells, respectively ( Fig. 3d ). In HeLa cells, SMAD7 overexpression reduced biotin-labelled TβRI level, whereas NR4A1 co-expression inhibited SMAD7 expression and restored the membrane-associate TβRI level ( Fig. 3e ). Furthermore, we found that NR4A1-deficient MEFs showed higher expression levels and longer half-lives of SMAD7 than wild-type MEFs ( Fig. 3f ). When we restored NR4A1 expression in NR4A1-deficient cells, SMAD7 expression was decreased and SMAD7 degradation was accelerated ( Fig. 3g ). As expected, in NR4A1-depleted cells, SMAD7 polyubiquitination was strongly diminished ( Supplementary Fig. 4b ). NR4A1 and SMAD7 co-localized in the nucleus, but only in the presence of MG132. Ectopic-expressed SMAD7 was degraded in HaCaT cells that stably expressed NR4A1; only in a few cells some cytoplasmic SMAD7 remained ( Supplementary Fig. 4c ). These results together suggest that NR4A1 potentiates TGF-β/SMAD signalling by facilitating SMAD7 degradation. 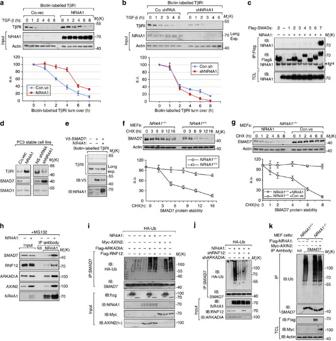Figure 3: NR4A1 interacts and promotes AXIN2–RNF12/ARKADIA complex-mediated SMAD7 degradation. (a,b) Immunoblot analysis of biotinylated TβRI in MDA-MB-231 cells infected with lentivirus expressing (a) or knocking down (b) NR4A1 and treated with TGF-β (5 ng ml−1) for the indicated time points. Co.vec, control empty vector. Co.shRNA, non-targeting shRNA (n=3). Band intensity was normalized to thet=0 controls. Results are shown as means±s.d. of three independent sets of experiments. (c) Immunoblot analysis of immunoprecipitation (IP) samples from HEK293T cells transfected with Flag-SMADs (1–7) and NR4A1 plasmids as indicated. (d) Immunoblot analysis of TβRI and SMAD7 in PC3 cells stably expressing NR4A1 or in which NR4A1 is depleted. SMAD1 immunoblot was taken along as a loading control. (e) Immunoblot (IB) analysis of biotinylated TβRI in HeLa cells transfected with V5-SMAD7 and NR4A1. (f) Immunoblot analysis of SMAD7 expression inNR4A1+/+andNR4A1−/−MEFs treated with cycloheximide (CHX, 20 μg ml−1) for the indicated time points (n=3). (g) Restoration of the expression of NR4A1 inNR4A1−/−MEFs re-established the faster degradation rates of SMAD7 as observed in wild-type MEFs (n=3). Forfandg, Band intensity was normalized to thet=0 controls. Results are shown as means ±s.d. of three independent sets of experiments. (h) HEK293T cells transfected with or without NR4A1 were treated with MG132 (5 μM) overnight and lysed for IP with NR4A1 antibody followed by immunoblot analysis. (i) HEK293T cells infected with lentivirus expressing NR4A1, AXIN2, ARKADIA and RNF12 were treated with MG132 (5 μM) overnight and lysed for the ubiquitination assay followed by immunoblot analysis. (j) HEK293T cells infected with lentivirus expressing NR4A1, RNF12 targeting shRNA (shRNF12) and/or ARKADIA targeting shRNA (shARKADIA) were treated with MG132 (5 μM) overnight and lysed for the ubiquitination assay followed by immunoblot analysis. (k)NR4A1+/+andNR4A1−/−primary MEF cells infected with Flag-NR4A1 or HA-AXIN2 lentivirus were treated with MG132 (5 μM) overnight and lysed for ubiquitination assay followed by immunoblot analysis. Ub, ubiquitin. Figure 3: NR4A1 interacts and promotes AXIN2–RNF12/ARKADIA complex-mediated SMAD7 degradation. ( a , b ) Immunoblot analysis of biotinylated TβRI in MDA-MB-231 cells infected with lentivirus expressing ( a ) or knocking down ( b ) NR4A1 and treated with TGF-β (5 ng ml −1 ) for the indicated time points. Co.vec, control empty vector. Co.shRNA, non-targeting shRNA ( n =3). Band intensity was normalized to the t =0 controls. Results are shown as means±s.d. of three independent sets of experiments. ( c ) Immunoblot analysis of immunoprecipitation (IP) samples from HEK293T cells transfected with Flag-SMADs (1–7) and NR4A1 plasmids as indicated. ( d ) Immunoblot analysis of TβRI and SMAD7 in PC3 cells stably expressing NR4A1 or in which NR4A1 is depleted. SMAD1 immunoblot was taken along as a loading control. ( e ) Immunoblot (IB) analysis of biotinylated TβRI in HeLa cells transfected with V5-SMAD7 and NR4A1. ( f ) Immunoblot analysis of SMAD7 expression in NR4A1 +/+ and NR4A1 −/− MEFs treated with cycloheximide (CHX, 20 μg ml −1 ) for the indicated time points ( n =3). ( g ) Restoration of the expression of NR4A1 in NR4A1 −/− MEFs re-established the faster degradation rates of SMAD7 as observed in wild-type MEFs ( n =3). For f and g , Band intensity was normalized to the t =0 controls. Results are shown as means ±s.d. of three independent sets of experiments. ( h ) HEK293T cells transfected with or without NR4A1 were treated with MG132 (5 μM) overnight and lysed for IP with NR4A1 antibody followed by immunoblot analysis. ( i ) HEK293T cells infected with lentivirus expressing NR4A1, AXIN2, ARKADIA and RNF12 were treated with MG132 (5 μM) overnight and lysed for the ubiquitination assay followed by immunoblot analysis. ( j ) HEK293T cells infected with lentivirus expressing NR4A1, RNF12 targeting shRNA (shRNF12) and/or ARKADIA targeting shRNA (shARKADIA) were treated with MG132 (5 μM) overnight and lysed for the ubiquitination assay followed by immunoblot analysis. ( k ) NR4A1 +/+ and NR4A1 −/− primary MEF cells infected with Flag-NR4A1 or HA-AXIN2 lentivirus were treated with MG132 (5 μM) overnight and lysed for ubiquitination assay followed by immunoblot analysis. Ub, ubiquitin. Full size image SMAD7 is targeted for degradation by E3 ligases ARKADIA, RNF12 and also by AXIN1 (refs 8 , 9 , 20 , 21 , 22 ). We found that AXIN2 could also interact with endogenous ARKADIA, RNF12 and rely on them to target SMAD7 for polyubiquitination ( Supplementary Fig. 4d,e ). Immunoprecipitation studies showed that NR4A1 associated with the SMAD7/ARKADIA/RNF12/AXIN2 complex endogenously but not with SMURFs ( Fig. 3h ). Importantly, as a scaffold protein for the SMAD7 destruction complex, endogenous AXIN2 (but not AXIN1 ) expression was sharply upregulated by NR4A1 ( Fig. 3h ). SMAD7 polyubiquitination was increased by ectopic NR4A1 expression. Co-expression of NR4A1 or AXIN2 with ARKADIA or RNF12 synergistically enhanced the polyubiquitination of SMAD7 ( Fig. 3i ). Depletion of E3 ligase RNF12 or ARKADIA mitigated the SMAD7 polyubiquitination. Double depletion of RNF12 and ARKADIA decreased SMAD7 polyubiquitination to a basal level, indicating that NR4A1 enhances SMAD7 polyubiquitination mainly via both E3 ligases RNF12 and ARKADIA ( Fig. 3j ). Moreover, polyubiquitinated SMAD7 accumulated in NR4A1 +/+ MEFs but was undetectable in NR4A1 −/− cells, although it was detected again on restoring the expression of NR4A1 or on overexpression of AXIN2 ( Fig. 3k ). Depleting AXIN2 greatly decreased NR4A1-triggered endogenous SMAD7 polyubiquitination, suggesting that NR4A1 relies on the E3 ubiquitin ligase RNF12/ARKADIA and scaffold protein AXIN2 to degrade SMAD7. NR4A1 directly induces AXIN2 To explore the mechanism by which NR4A1 induces AXIN2, we first examined the endogenous AXIN2 protein expression in different mouse or human cell lines stably expressing NR4A1. AXIN2 was upregulated in mouse NMuMG and human HaCaT or PC3 cells ( Fig. 4a ). The AXIN2 protein level was lower in primary NR4A1 −/− MEFs than in control MEFs ( Fig. 4b ). The real-time quantitative (qRT)–PCR analysis showed that stable NR4A1 expression in HaCaT, PC3, NMuMG and HEK293T cells dramatically increased AXIN2 mRNA levels, whereas NR4A1 depletion decreased the mRNA level to roughly 50% ( Fig. 4c,d and Supplementary Fig. 5a ). In NR4A1 −/− MEFs, the level of AXIN2 mRNA was 60% lower than the level in wild-type MEFs ( Fig. 4e ). 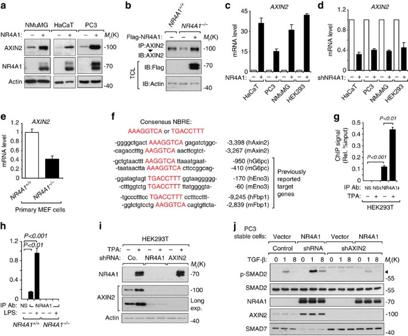Figure 4: NR4A1 directly induces AXIN2 expression. (a) Immunoblot analysis of AXIN2 and NR4A1 in HaCaT, NMuMG and PC3 cells stably expressing NR4A1 or control cells. Actin was included as a loading control. (b)NR4A1+/+andNR4A1−/−MEFs infected with or without Flag-NR4A1 lentivirus were lysed for immunoprecipitation (IP) with AXIN2 antibody followed by immunoblot. (c,d) qRT–PCR analysis ofAXIN2in HaCaT, PC3, NMuMG and HEK293T cells stably expressing NR4A1 (c) or depleted of NR4A1 (d). The mRNA level in the control was set to ‘1’ for each cell type (n=3). (e) qRT–PCR ofAXIN2inNR4A1+/+andNR4A1−/−MEFs. Data are presented as mean±s.d. (n=3). (f) Sequences and locations of putative NGFI-B-response elements (NBRE) in human and mouseAXIN2promoters and identified gluconeogenic genes24. (g,h) ChIP in HEK293T cells treated with or without 100 ng ml−1TPA (g) or inNR4A1+/+andNR4A1−/−MEFs treated with or without 2 μg ml−1lipopolysaccharide for 4 h (h). Data represent mean±s.d.n=3.P<0.01 orP<0.001 by Student’st-test. (i) Immunoblot of NR4A1 and AXIN2 in HEK293T cells with NR4A1 or AXIN2 depletion by lentiviral infection and induced with 100 ng ml−112-O-tetradecanoylphorbol-13-acetate (TPA) for 4 h. Co., non-targeting shRNA. Actin was included as a loading control. (j) PC3 cells infected with empty vector, NR4A1, control shRNA or AXIN2 shRNA as indicated were treated with TGF-β (5 ng ml−1) for the indicated time and then lysed for immunoblot analysis. Figure 4: NR4A1 directly induces AXIN2 expression. ( a ) Immunoblot analysis of AXIN2 and NR4A1 in HaCaT, NMuMG and PC3 cells stably expressing NR4A1 or control cells. Actin was included as a loading control. ( b ) NR4A1 +/+ and NR4A1 −/− MEFs infected with or without Flag-NR4A1 lentivirus were lysed for immunoprecipitation (IP) with AXIN2 antibody followed by immunoblot. ( c , d ) qRT–PCR analysis of AXIN2 in HaCaT, PC3, NMuMG and HEK293T cells stably expressing NR4A1 ( c ) or depleted of NR4A1 ( d ). The mRNA level in the control was set to ‘1’ for each cell type ( n =3). ( e ) qRT–PCR of AXIN2 in NR4A1 +/+ and NR4A1 −/− MEFs. Data are presented as mean±s.d. ( n =3). ( f ) Sequences and locations of putative NGFI-B-response elements (NBRE) in human and mouse AXIN2 promoters and identified gluconeogenic genes [24] . ( g , h ) ChIP in HEK293T cells treated with or without 100 ng ml −1 TPA ( g ) or in NR4A1 +/+ and NR4A1 −/− MEFs treated with or without 2 μg ml −1 lipopolysaccharide for 4 h ( h ). Data represent mean±s.d. n =3. P <0.01 or P <0.001 by Student’s t -test. ( i ) Immunoblot of NR4A1 and AXIN2 in HEK293T cells with NR4A1 or AXIN2 depletion by lentiviral infection and induced with 100 ng ml −1 12- O -tetradecanoylphorbol-13-acetate (TPA) for 4 h. Co., non-targeting shRNA. Actin was included as a loading control. ( j ) PC3 cells infected with empty vector, NR4A1, control shRNA or AXIN2 shRNA as indicated were treated with TGF-β (5 ng ml −1 ) for the indicated time and then lysed for immunoblot analysis. Full size image NR4A1 was previously identified as a transcription factor consisting of an amino-terminal transactivation domain (TA), a DNA-binding domain with two zinc fingers, and a carboxy-terminal ligand-binding domain [23] . NR4A1 has been shown to activate target genes via the specific NGFI-B-response element in their promoters [11] , [24] . Both TA and DNA-binding domain of NR4A1 are required for AXIN2 mRNA induction, as deletion of either domain (dTA and d260-340, respectively) eliminates such response ( Supplementary Fig. 5b ). We then analysed AXIN2 promoter sequences and found a putative NR4A1-binding site in both the human and mouse AXIN2 promoters ( Fig. 4f ). Chromatin immunoprecipitation (ChIP) assays in HEK293T, HaCaT, PC3 and NMuMG cells stably expressing Flag-NR4A1 demonstrated strong NR4A1 binding to the AXIN2 promoter ( Supplementary Fig. 5c,d ). NR4A1 can be quickly and potently induced by 12- O -tetradecanoylphorbol-13-acetate (TPA) or lipopolysaccharide depending on the cell type [11] , [25] . Challenging HEK293T cells with TPA potently enhanced the binding of endogenous NR4A1 to the AXIN2 promoter ( Fig. 4g ). The addition of lipopolysaccharide increased endogenous NR4A1 binding to the AXIN2 promoter in wild-type, but not NR4A1 −/− MEFs ( Fig. 4h ). These results indicated that AXIN2 is a direct target gene of NR4A1. Consistent with the ChIP results, TPA promoted AXIN2 protein expression in control, but not in NR4A1-depleted cells ( Fig. 4i ). To explore whether NR4A1-activated TGF-β/SMAD signalling is dependent on the induction of AXIN2, we knocked down AXIN2 in NR4A1-PC3 cells. We found that phospho-SMAD2 decreased on AXIN2 depletion, at both basal and NR4A1-stimulated levels, and inversely correlated with SMAD7 protein expression ( Fig. 4j ). However, on ectopic expression we found that AXIN2 is weaker than NR4A1 in promoting the TGF-β-induced transcriptional response, and that NR4A1 depletion weakly but significantly attenuated the AXIN2-induced SMAD3/SMAD4 response. Taken together, the results indicate that NR4A1 directly induces AXIN2 expression, both NR4A1 and AXIN2 form part of the destruction complex, which promotes SMAD7 degradation, thereby potentiating TGF-β/SMAD signalling. NR4A1 promotes TGF-β-induced EMT TGF-β stimulates epithelial-to-mesenchymal transition (EMT), cell migration, invasion and metastasis of breast cancer cells [26] , [27] . EMT is a process by which cells undergo a morphological switch from the epithelial polarized phenotype to the mesenchymal fibroblastoid phenotype. At the molecular level, EMT is defined by the loss of cell–cell adhesion molecules (for example, E-cadherin and ZO-1), downregulation of epithelial differentiation markers including cytokeratins and E-cadherin and transcriptional induction of mesenchymal markers such as vimentin, fibronectin and N-cadherin [28] . HaCaT cells stably expressing NR4A1 showed an obvious morphological change from an epithelial to a mesenchymal cell shape ( Fig. 5a ). Immunofluorescence and immunoblotting further showed that ectopic expression of NR4A1 potentiated TGF-β-induced changes in EMT marker expression ( Fig. 5b and Supplementary Fig. 6a,d,e ). Conversely, depletion of NR4A1 attenuated these TGF-β-induced effects ( Fig. 5c and Supplementary Fig. S6b,c ). Of note, treatment with SB431542 mitigated the effect of NR4A1 on EMT ( Fig. 5d ), indicating that NR4A1 promotes EMT by cooperating with basal TGF-β signalling. Furthermore, we observed a weak but significant positive correlation between NR4A1 and mesenchymal markers in clinical samples from breast cancer patients ( Fig. 5e ). Taken together, these results indicate that NR4A1 is an important enhancer for TGF-β-induced EMT. 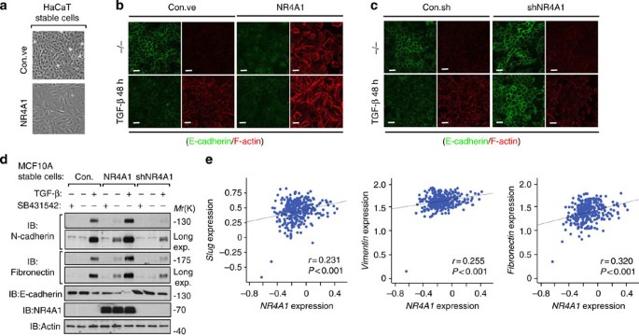Figure 5: NR4A1 promotes TGF-β-induced EMT and is associated with bad prognosis in breast cancer patients. (a) Light image of HaCaT cells stably expressed with empty vector (Con.ve) or NR4A1. (b,c) Immunofluorescence of HaCaT cells stably expressing NR4A1 (b) or with knockdown of NR4A1 (c) and treated with or without TGF-β (5 ng ml−1) for 48 h. Scale bar, 20 μm. (d) Immunoblot analysis of MCF10A cells stably expressing or with knockdown of NR4A1 and treated with TGF-β (5 ng ml−1) and SB431542 (10 μM) for 48 h. Actin immunoblot has been used as a loading control. (e) Scatter plot showing the positive correlation betweenNR4A1andSlug/Vimentin/Fibronectinexpression in the NKI295 patients’ clinical data set (n=295). Pearson’s coefficient tests were performed to assess statistical significance. Figure 5: NR4A1 promotes TGF-β-induced EMT and is associated with bad prognosis in breast cancer patients. ( a ) Light image of HaCaT cells stably expressed with empty vector (Con.ve) or NR4A1. ( b , c ) Immunofluorescence of HaCaT cells stably expressing NR4A1 ( b ) or with knockdown of NR4A1 ( c ) and treated with or without TGF-β (5 ng ml −1 ) for 48 h. Scale bar, 20 μm. ( d ) Immunoblot analysis of MCF10A cells stably expressing or with knockdown of NR4A1 and treated with TGF-β (5 ng ml −1 ) and SB431542 (10 μM) for 48 h. Actin immunoblot has been used as a loading control. ( e ) Scatter plot showing the positive correlation between NR4A1 and Slug / Vimentin / Fibronectin expression in the NKI295 patients’ clinical data set ( n =295). Pearson’s coefficient tests were performed to assess statistical significance. Full size image NR4A1 and TβRI are required for the metastasis Next we analysed the role of NR4A1 in TGF-β-induced breast cancer cell migration in the context of biologically (or oncogenically) relevant extracellular cues. NR4A1 knockdown attenuated TGF-β-induced migration in breast cancer MDA-MB-231 cells ( Fig. 6a–c ). Notably, the TGF-β-induced expression of osteolytic cytokine interleukin 11 ( IL-11 ) and EMT inducer (and repressor of E-cadherin) SNAIL was suppressed in NR4A1-depleted MDA-MB-231 cells ( Fig. 6d,e ). 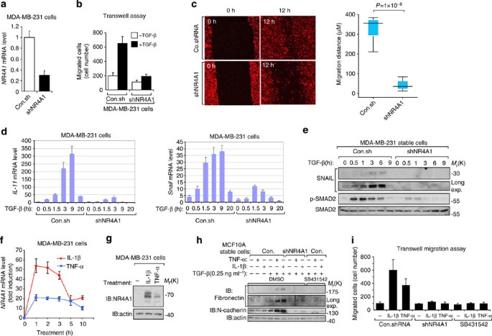Figure 6: Inflammatory cytokines-induced NR4A1 promote TGF-β-induced responses, including cell migration. (a) qRT–PCR analysis of NR4A1 depletion efficiency in MDA-MB-231 cells. (b) NR4A1 depletion inhibits TGF-β-induced migration. Migrated cells were counted from four random fields, and means±s.d. were calculated in Student’st-tests (P<0.05,n=3). (c) Control and NR4A1-depleted MDA-MB-231/mcherry cells were scraped in a straight line to create a ‘scratch’ with a p200 pipette tip. Cells were treated with TGF-β (5 ng ml−1). Images were taken under the fluorescence microscopy at time 0 and 12 h. The distances between one side of scratch and other were measured.n=12 for each experimental group; the horizontal line in the middle of each box indicates the median (50th percentile), the top and bottom borders of the box mark the 75th and 25th percentiles, and the whiskers mark the 90th and 10th percentiles.P<0.001 by Student’st-test. (d) qRT–PCR analysis of control (Con.sh) and MDA-MB-231 cells stably depleted of NR4A1 (shNR4A1) and treated with TGF-β (5 ng ml−1) for indicated time points. Data are presented as mean±s.d. (n=3). (e) Immunoblot analysis of control (Con.sh) or MDA-MB-231 cells with stably knockdown of NR4A1 (shNR4A1) and treated with TGF-β (5 ng ml−1) for indicated time points. (f) qRT–PCR analysis of MDA-MB-231 cells treated with IL-1β (10 ng ml−1) or TNF-α (10 ng ml−1) for indicated time points. Data are presented as mean±s.d. (n=3). (g) Immunoblot of MDA-MB-231 cells treated with or without IL-1β (10 ng ml−1) and TNF-α (10 ng ml−1) for 2 h. (h) Immunoblot (IB) of control (Con.) or MCF10A-Ras cells stably depleting NR4A1 (shNR4A1) and treated with IL-1β (10 ng ml−1), TNF-α (10 ng ml−1), TGF-β (0.25 ng ml−1) and SB431542 (10 μM) as indicated for 48 h. (i) Transwell migration assay of control or MDA-MB-231 cells stably depleted of NR4A1 (shNR4A1) and treated with or without IL-1β (10 ng ml−1), TNF-α (10 ng ml−1) and SB431542 (10 μM) as indicated for 8 h. Migrated cells were counted from four random fields, and means±s.d. were calculated in Student’st-tests (P<0.05,n=3). Figure 6: Inflammatory cytokines-induced NR4A1 promote TGF-β-induced responses, including cell migration. ( a ) qRT–PCR analysis of NR4A1 depletion efficiency in MDA-MB-231 cells. ( b ) NR4A1 depletion inhibits TGF-β-induced migration. Migrated cells were counted from four random fields, and means±s.d. were calculated in Student’s t -tests ( P <0.05, n =3). ( c ) Control and NR4A1-depleted MDA-MB-231/mcherry cells were scraped in a straight line to create a ‘scratch’ with a p200 pipette tip. Cells were treated with TGF-β (5 ng ml −1 ). Images were taken under the fluorescence microscopy at time 0 and 12 h. The distances between one side of scratch and other were measured. n =12 for each experimental group; the horizontal line in the middle of each box indicates the median (50th percentile), the top and bottom borders of the box mark the 75th and 25th percentiles, and the whiskers mark the 90th and 10th percentiles. P <0.001 by Student’s t -test. ( d ) qRT–PCR analysis of control (Con.sh) and MDA-MB-231 cells stably depleted of NR4A1 (shNR4A1) and treated with TGF-β (5 ng ml −1 ) for indicated time points. Data are presented as mean±s.d. ( n =3). ( e ) Immunoblot analysis of control (Con.sh) or MDA-MB-231 cells with stably knockdown of NR4A1 (shNR4A1) and treated with TGF-β (5 ng ml −1 ) for indicated time points. ( f ) qRT–PCR analysis of MDA-MB-231 cells treated with IL-1β (10 ng ml −1 ) or TNF-α (10 ng ml −1 ) for indicated time points. Data are presented as mean±s.d. ( n =3). ( g ) Immunoblot of MDA-MB-231 cells treated with or without IL-1β (10 ng ml −1 ) and TNF-α (10 ng ml −1 ) for 2 h. ( h ) Immunoblot (IB) of control (Con.) or MCF10A-Ras cells stably depleting NR4A1 (shNR4A1) and treated with IL-1β (10 ng ml −1 ), TNF-α (10 ng ml −1 ), TGF-β (0.25 ng ml −1 ) and SB431542 (10 μM) as indicated for 48 h. ( i ) Transwell migration assay of control or MDA-MB-231 cells stably depleted of NR4A1 (shNR4A1) and treated with or without IL-1β (10 ng ml −1 ), TNF-α (10 ng ml −1 ) and SB431542 (10 μM) as indicated for 8 h. Migrated cells were counted from four random fields, and means±s.d. were calculated in Student’s t -tests ( P <0.05, n =3). Full size image NR4A1 is an immediate early response gene of which the expression is low in most non-stimulated cells. To obtain clues for the (patho) physiological function of NR4A1, we examined various interstitial cytokines and related agents for their effects on NR4A1 expression in breast cancer cells. Among these agents, IL-1β and tumour necrosis factor-α (TNF-α) strongly induced NR4A1 expression ( Fig. 6f,g ). This is consistent with previous report in which nuclear factor-κB activation by inflammatory stimuli was reported to induce NR4A1 (ref. 25 ). Interestingly, we found that in clinical breast cancer samples, NR4A1 levels correlated with IL-1β and TNF-α expression, but not with other inflammatory cytokines ( Supplementary Fig. 7a,b ). Moreover, in MCF10A-Ras cells, co-treatment with IL-1β/TNF-α potentiated the TGF-β-induced EMT changes and these effects were blocked by TβRI kinase inhibitor SB431542 or NR4A1 depletion ( Fig. 6h ). We also found that the migration of MDA-MB-231 cells was promoted by IL-1β or TNF-α, which was blocked by SB431542 or NR4A1 knockdown ( Fig. 6i ). Thus, either IL-1β or TNF-α is likely to promote TGF-β-mediated EMT and migration by stimulating NR4A1 expression. We subsequently investigated the role of NR4A1 in breast cancer metastasis. The metastasis of MDA-MB-231 cells in xenograft models was found to be dependent on TGF-β receptor signalling in tumour cells [29] , [30] , [31] . We selected stable MDA-MB-231 cells that ectopically expressed NR4A1 to an amount equivalent to inflammatory cytokine-induced level. In vivo intracardial injection of these cells showed that ectopic expression of NR4A1 strongly potentiated the bone colonization of circulating MDA-MB-231 cells, and this effect could be blocked by pretreatment of cells with SB431542 ( Fig. 7a–c ). Moreover, whereas IL-1β pretreatment potentiated the metastasis, NR4A1 depletion blocked both the basal and IL-1β-induced metastasis in mice ( Fig. 7d–f ). These results were further validated using a zebrafish xenograft model. We found that the invasion and metastasis of MDA-MB-231 cells in zebrafish were inhibited when NR4A1 was depleted ( Supplementary Fig. 8a–e ). Moreover, fully consistent with our mouse data, invasion and metastasis triggered by IL-1β or TNF-α pretreatment were repressed on NR4A1 knockdown ( Supplementary Fig. 8f–j ). These results suggest that inflammatory cytokines regulate invasion and metastasis of breast cancer cells, at least partially, via a NR4A1-TGF-β/SMAD signalling cascade-dependent manner. 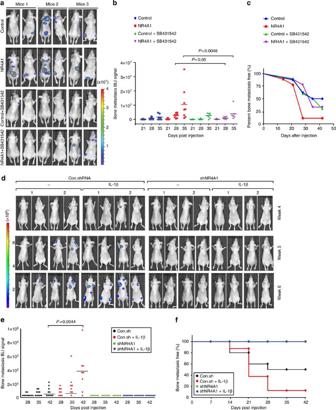Figure 7: Inflammatory cytokines promote TGF-β-induced EMT/migration andin vivoinvasion/metastasis in a NR4A1-dependent manner. (a–c) Bioluminescent imaging (BLI) of three representative mice from each group at week 5 injected with control or MDA-MB-231 cells stably infected with NR4A1 and pretreated with or without SB431542 (10 μM) for 16 h. Both ventral and dorsal images are shown (a). BLI signal of every mouse (b) and the percentage of bone metastasis-free mice (c) in each experimental group was followed in time and are shown. (d–f) BLI of two representative mice from each group at weeks 4, 5 and 6 injected with control or MDA-MB-231 cells stably depleted of NR4A1 and pretreated with or without IL-1β (10 ng ml−1) for 6 h. Both ventral and dorsal images are shown (d). BLI signal of every mouse (e) and the percentage of bone metastasis-free mice (calculated in Student’st-tests) (f) in each experimental group was followed in time and are shown. Figure 7: Inflammatory cytokines promote TGF-β-induced EMT/migration and in vivo invasion/metastasis in a NR4A1-dependent manner. ( a – c ) Bioluminescent imaging (BLI) of three representative mice from each group at week 5 injected with control or MDA-MB-231 cells stably infected with NR4A1 and pretreated with or without SB431542 (10 μM) for 16 h. Both ventral and dorsal images are shown ( a ). BLI signal of every mouse ( b ) and the percentage of bone metastasis-free mice ( c ) in each experimental group was followed in time and are shown. ( d – f ) BLI of two representative mice from each group at weeks 4, 5 and 6 injected with control or MDA-MB-231 cells stably depleted of NR4A1 and pretreated with or without IL-1β (10 ng ml −1 ) for 6 h. Both ventral and dorsal images are shown ( d ). BLI signal of every mouse ( e ) and the percentage of bone metastasis-free mice (calculated in Student’s t -tests) ( f ) in each experimental group was followed in time and are shown. Full size image NR4A1 correlates with SMAD activation and poor prognosis In light of our observations, we analysed the potential pathological role of NR4A1 in breast cancer patients. Given the fact that inflammatory cytokines could induce NR4A1 and promote metastasis in animal invasion/metastasis models, we compared the NR4A1 expression in a clinical data set of breast cancer patients with high versus low lymphocyte infiltration. Samples with high infiltration have elevated NR4A1 expression ( Supplementary Fig. 9a ). Notably, high infiltration also correlates with a poor prognosis ( Supplementary Fig. 9b ) and shorter lifespan ( Supplementary Fig. 9c ). To further confirm the effect of NR4A1 in human breast cancer, we performed an immunohistochemical analysis of a tissue microarray (TMA) containing samples from 175 breast cancer patients and found a statistically significant inverse correlation between the NR4A1 expression and the relapse-free survival during 200 months ( Fig. 8a and Supplementary Table 1 ). Consistent with this result, mining of a publicly available data set of breast cancer patients revealed that up to about 14% of patients had gained NR4A1 mRNA expression (with gene amplification playing a minor role; Supplementary Fig. 9d ), and that there is a trend towards poor prognosis for patients with elevated NR4A1 expression ( Supplementary Fig. 9e ). Moreover, when we compared by immunohistochemical analysis NR4A1 and p-SMAD2 expression levels in the breast cancer TMA, we found a statistically significant correlation between their expression ( Fig. 8b,c ). The correlation is weak, which is not so surprising as the p-SMAD2 level is subject to regulation by many different stimuli. Thus, NR4A1 may regulate in part TGF-β/SMAD signalling activity in human breast cancer. Taken together, our findings suggest that the inflammation, via the induction of NR4A1, participates in the cancer progression via TGF-β/SMAD activation. 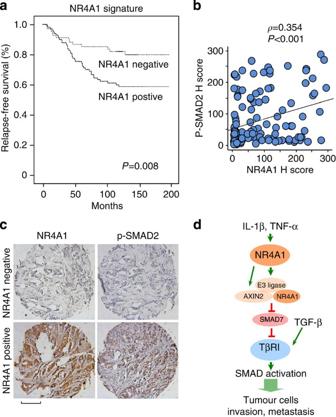Figure 8: NR4A1 correlates with poor prognosis in breast cancer patients. (a) Kaplan–Meier curves showing that the relapse-free survival of individuals with NR4A1 expression is significantly lower than those without NR4A1 expression (P=0.008) by log-rank test. (b) Graph showing the correlation between NR4A1 expression levels and those of p-SMAD2 in TMAs from 175 samples from individuals with breast cancer. Not all spots were evaluable in all stainings. A Spearman’s test was used, and the correlation coefficient (Spearman’sρ=0.354) and the two-tailed significance (P<0.001) are shown. (c) Representative images of NR4A1 and p-SMAD2 immunohistochemistry results are shown (scale bar, 50 μm). (d) Working model of NR4A1 in regulating TGF-β/SMAD signalling in breast cancer. Figure 8: NR4A1 correlates with poor prognosis in breast cancer patients. ( a ) Kaplan–Meier curves showing that the relapse-free survival of individuals with NR4A1 expression is significantly lower than those without NR4A1 expression ( P =0.008) by log-rank test. ( b ) Graph showing the correlation between NR4A1 expression levels and those of p-SMAD2 in TMAs from 175 samples from individuals with breast cancer. Not all spots were evaluable in all stainings. A Spearman’s test was used, and the correlation coefficient (Spearman’s ρ =0.354) and the two-tailed significance ( P <0.001) are shown. ( c ) Representative images of NR4A1 and p-SMAD2 immunohistochemistry results are shown (scale bar, 50 μm). ( d ) Working model of NR4A1 in regulating TGF-β/SMAD signalling in breast cancer. Full size image The extracellular cytokine TGF-β and nuclear orphan receptor NR4A1 are of key importance in maintaining cellular homoeostasis. Perturbation in TGF-β and NR4A1 signalling has been implicated in cancer, and for both factors tumour suppressive and promoting activities have been reported. In this paper, we have linked these two multifunctional signalling components and elucidated the molecular mechanism by which NR4A1 strongly activates TGF-β/SMAD signalling, and have investigated the biological consequences of this interplay in breast cancer invasion and metastasis via inflammatory cytokines ( Fig. 8d ). NR4A1, of which the expression is regulated by many stimuli, has been implicated as a key regulator of a wide range of pathophysiological responses including tumorigenesis, inflammation, glucose and lipid homoeostasis, adipogenesis and vascular remodelling. However, the underlying mechanism of which NR4A1 elicits its multifunctional effects is not yet fully understood. Here through the functional genetic screens, we identified NR4A1 as a strong TGF-β signalling activator. NR4A1 potently promotes TGF-β/SMAD activation in different cultured cells, while TGF-β-SMAD signalling was impaired in NR4A1 knockout and knockdown cells. Ectopic NR4A1 expression in mouse liver induced endogenous SMAD2 phosphorylation in situ . Moreover, cells with ectopic NR4A1 expression that were injected into mice demonstrated a dramatic higher SMAD3/4 transcriptional activity. Mechanistically, NR4A1 functions as a destruction scaffold for inhibitory SMAD7 by recruiting AXIN2 and E3 ubiquitin ligases RNF12 or ARKADIA. In addition, NR4A1, by acting as a strong direct transcriptional inducer for AXIN2 (but not AXIN1 ), compensates the limiting pool of oncogenic AXIN2 (ref. 32 ) and ( Supplementary Fig. 6f–h ), thereby enforcing SMAD7 degradation. Our data that AXIN2 interacts with and stimulates SMAD7 degradation and thereby sensitizes cells to TGF-β are in contrast with report that AXIN1 associates with SMAD3 and mediates its GSK3β-dependent degradation [33] . AXIN2, but not AXIN1, was found to be potently induced by NR4A1. Thus, AXIN isoforms may differentially affect TGF-β signalling. NR4A1-mediated downregulation of SMAD7 prolonged active TβRI levels on the plasma membrane, and led to more intense and sustained SMAD signalling. Functionally, NR4A1 potently promotes TGF-β-induced EMT and cell migration. Endogenous NR4A1 was found to be required for breast cancer invasion and metastasis. NR4A2 and NR4A3, the family members of NR4A1, also respond weakly to the stimulation of IL-1β/TNF-α and participate in TGF-β/SMAD signal activation, but less potently ( Supplementary Fig. 6i,j ). The reason for NR4A2 and 3 to be less active in promoting TGF-β/SMAD signalling requires further investigation. As NR4A1 controls TβRI levels, it is possible that NR4A1 may also potentiate TGF-β/TβRI-mediated tumour suppressive effects, including its cytostatic effects on normal and premalignant cells. An interesting area of research will therefore be the interplay between NR4A1 and TGF-β signalling and their biphasic roles in tumour progression. More and more evidence indicate that immune cells, including inflammatory cells, have tumour-promoting activity. Indeed, many cancers arise from sites of infection, chronic irritation and inflammation [34] . During tumour progression, immune cells similar to monocytes, neutrophils, regulatory T cells and myeloid-derived suppressor cells are attracted to tumours where they secrete various cytokines that participate in the neoplastic process fostering proliferation, survival and migration [34] , [35] . We show here that, in aggressive breast cancer cells, NR4A1 expression is potently induced by inflammatory cytokines IL-1β or TNF-α. Consistent with this notion, we found that NR4A1 expression is elevated in breast cancer patients with high immune infiltration. We also demonstrated that pretreatment of breast cancer cells with IL-1β, in an NR4A1-dependent manner, promoted TGF-β-mediated breast cancer progression using zebrafish and mouse models. Using breast cancer TMA and mining of publicly available data sets, we found that NR4A1 expression is correlated with poor prognosis of breast cancer patients. Our results are consistent with the emerging role for nuclear factor-κβ activation by inflammatory cytokines, such as TNFα, as promotor and accelerator of TGF-β-driven tumour progression [36] , [37] . In contrast to our data in which NR4A1 stimulates SMAD7 degradation, interferon-γ via a JAK1/STAT1-mediated pathway has been shown to induce SMAD7 expression [38] , but this response is mainly linked with anti-tumour immune effects [39] . Taken together, our results have revealed a new mechanism by which the microenvironment stimulates breast cancer cell invasion and metastasis. Clinical trials for TGF-β targeting agents for anti-cancer therapy have been initiated. The ability of NR4A1 to hyperactivate the pro-oncogenic effects of TGF-β could make it a biomarker of response to anti-TGF-β therapy of advanced breast cancer. In addition, inhibitors of NR4A1 function may have therapeutic potential in cancer and other diseases. As NR4A1 and TGF-β have critical roles in a wide spectrum of normal developmental and homoeostatic processes and many pathological conditions, our results may have broad implications. Mice and cell culture Primary mouse embryo fibroblasts (MEFs) from wild-type and NR4A1 −/− mice on a C57BL/6 background [40] (kindly provided by B.R. Binder (Vienna, Austria) were collected at E9.5, disaggregated enzymatically in trypsin (10 min at room temperature) and plated. Human cervical cancer HeLa cell line, human prostate cancer PC3 cell line, breast cancer Namru Mouse Mammary Gland NMuMG cell line, human MDA-MB-231 cell line and human MCF10A-RAS-transformed cell line, human HaCAT keratinocyte cell line, human HN5 cell line and primary MEFs were cultured in DMEM supplemented with 10% FBS (Hyclone) and 100 U ml −1 penicillin/streptomycin (Invitrogen). All cell lines were obtained from American Tissue Culture Collection, except for MEFs and MCF10A-RAS-transformed cell line. MEFs were isolated from wild-type and NR4A1 −/− mice as described above. MCF10A-RAS-transformed cell line was kindly provided by Dr Fred Miller (Barbara Ann Karmanos Cancer Institute, Detroit, MI, USA). Plasmids and reagents pLV-bc-CMV(puro)-Flag-NR4A1, pLV-bc-CMV(puro)-NR4A1 or pCMV-Myc-NR4A1 were amplified by PCR from pCMV-SPORT6 NR4A1 (Open Biosystems) and put into different expression vectors. pCMV-Myc-NR4A1dTA (d1-267aa) and pCMV-Myc-NR4A1d260-340 (aa) were amplified by PCR from pLV-bc-CMV-NR4A1 and cloned into pCMV-Myc vector. All of the constructs were verified by DNA sequencing. pCMV-HA-AXIN2 and pCMV-Flag-AXIN2 were kindly provided by Shengcai Lin of Xiamen University. 12- O -Tetradecanoylphorbol 13-acetate (TPA) and MG132 were purchased from Sigma. IL-1β and TNF-α were purchased from Pepro Tech. The antibodies used for immunoprecipitation, immunoblotting, immunofluorescence and ChIP were raised against the following proteins (dilution for western blot was shown): phospho-SMAD2 (Ser465/467) (#3101, Cell Signaling 1: 3,000), phospho-SMAD3 (a gift from Dr E. Leof, 1:3,000), SMAD2/3 (clone 18, BD Transduction Laboratories, 1:3,000), SMAD7 (N-19, sc-7004, Santa Cruz Biotechnology, 1:1,000), TβRI (sc-398, Santa Cruz Biotechnology, 1:1,000), β-actin (A5441, Sigma, 1:5,000), SMAD4 (B08, sc-7966, Santa Cruz Biotechnology, 1:1,000), c-Myc (a-14, sc-789, Santa Cruz Biotechnology, 1:1,000), HA (Y-11, sc-805, Santa Cruz Biotechnology, 1:1,000), Flag (M2, Sigma, 1:10,000), NR4A1(#3559, Cell Signaling, 1:3,000), AXIN2 (#2151, Cell Signaling for human cells (1:1,000) and a gift from Shengcai Lin for mouse cells (1:5,000) ), ARKADIA (B01P, Abnova, 1:1,000), RNF12 (clone 1G10, Abnova, 1:3,000), Ubiquitin (P4D1, Santa Cruz Biotechnology, 1:1,000), N-cadherin(610920, BD, 1:5,000), fibronectin (Sigma, 1:2,000) and E-cadherin (610181, BD, 1:5,000). Immunohistochemical staining and evaluation Primary antibodies to p-SMAD2 (1:50; Cell Signaling 3108), NR4A1 (1:200; Cell Signaling 3960) were used for immunohistochemical staining. The quantification of the staining was expressed as a H score. The H score was determined by the formula 3 × the percentage of strongly staining cells+2 × the percentage of moderately staining cells+the percentage of weakly staining cells, giving a range of 0–300 for the H scores. Patient selection The TMA analyses were performed on a TMA that was constructed from tumours that were diagnosed and treated in the Leiden University Medical Center (LUMC) between 1997 and 2003. Both percentage of positive cells and intensity was assessed and multiplied to calculate an H score. Relapse-free survival was defined as the time period between the incidence date and the occurrence of either locoregional or distant metastases (if applicable) or the last time the patient presented to the clinic for follow-up without invasive breast cancer disease. Mice adenoviral injection Adenovirus production and hepatic overexpression of NR4A1 in mouse liver was achieved by intravenous injection of recombinant adenovirus as described previously [41] . Full-length human NR4A1 cDNA (GenBank D49728) was inserted into replication-defective adenoviruses expressing cDNAs under control of the cytomegalovirus promoter. The adenoviruses were purified by CsCl gradient centrifugation. Animal care and experimental procedures were approved by the Animal Experimental Committee at LUMC. Male, 10–12 weeks old, C57Bl/6 mice ( n =6 per group; Charles River Laboratories, Wilmington, MA) were fed a standard chow diet (Special diet services, Essex, UK). Hepatic overexpression of NR4A1 in mouse liver was achieved by intravenous injection of recombinant adenovirus. Mice were killed 2 days after adenoviral treatment, after fasting for 4 h. The liver was dissected and part of the liver was fixed in formalin for immunohistochemical analysis, and the other part was used for RNA extraction. In vivo SMAD3/4 transcriptional activity assay Green fluorescence protein and NR4A1 overexpressing HN5 stable cells (5 × 10 6 ) were subcutaneously injected into nude mice. The same number of control HN5 and NR4A1 overexpressing HN5 cells were injected. The adenovirus for CAGA-Luc transcriptional reporter was added to the cells 24 h before injection. CAGA-Luc activity in xenograft HN5 cells expressing green fluorescence protein (left-hand-side xenograft) and NR4A1 (right-hand-side xenograft) was measured at time 0 (time of injection subcutaneously) and at time 48 h. During the experiment control, HN5 and NR4A1 overexpressing HN5 cells had similar growth rates. Experiments were performed three times. Immuno/transcriptional reporter assay Immunoprecipitation and immunoblot was performed as described previously [9] , [31] , [42] . Cells were lysed with 1 ml of lysis buffer (20 mM Tris–HCl, pH 7.4, 2 mM EDTA, 25 mM NaF, 1% Triton X-100) plus protease inhibitors (Sigma) for 10 min at 4 °C. After centrifugation at 12,000 g for 15 min, the protein concentration was measured and equal amounts of lysate were used in immunoprecipitations with different antibodies and protein A-Sepharose (GE Healthcare Bio-Sciences AB) for 3 h at 4 °C. Thereafter, the precipitants were washed three times with washing buffer (50 mM Tris–HCl, pH 8.0, 150 mM NaCl, 1% Nonidet P-40, 0.5% sodium deoxycholate and 0.1% SDS) and the immune complexes were eluted with sample buffer containing 1% SDS for 5 min at 95 °C. The immunoprecipitated proteins were then separated by SDS–polyacrylamide gel electrophoresis. Western blotting was performed with specific antibodies and secondary anti-mouse or anti-rabbit antibodies conjugated to horseradish peroxidase (Amersham Biosciences). Visualization was achieved with chemiluminescence. For reporter assay, cells were seeded in 24-well plates, and then transfected with the indicated plasmids. Twenty-four hours after transfection, cells were untreated or treated with TGF-β3 overnight. CAGA12-Luc was used as Smad3-Smad4-driven transcriptional reporter. Harvested cells were assayed for luciferase activity with a Perkin Elmer luminometer. The internal control, β-gal (30 ng) expression plasmid, was used to normalize transfection efficiency. Each experiment was performed in triplicate and data represent the mean±s.d. of three independent experiments after normalization to β-gal activity. Lentivirus transduction Lentiviruses were produced by co-transfecting pLKO-1 (for the shRNA knockdown) or pLV-bc-CMV (for cDNA expression) plasmids and helper plasmids pCMV-VSVG, pMDLg-RRE (gag/pol) and pRSV-REV into HEK293T cells. Cell supernatants were harvested 48 h after transfection and were used to infect cells or stored at −80 °C. To obtain stable cell lines, cells were infected at low confluence (20%) for 24 h with lentiviral supernatants diluted 1:1 with normal culture medium in the presence of 5 ng ml −1 polybrene (Sigma). Forty-eight hours after infection, cells were placed under puromycin selection for 1 week, and then passaged before use. Puromycin was used at 1 μg ml −1 to maintain selection pressure on stably transfected HaCaT, PC3, NMuMG, MCF10A-RAS and MDA-MB-231 cells. Lentiviral shRNAs were obtained from Sigma (MISSION shRNA). Typically, five shRNAs were identified, tested and the one or two most effective was used for the experiment. We used TRCN0000019426 for human NR4A1 knockdown, TRCN0000078540 for human AXIN2, TRCN0000004209 for human ARKADIA knockdown and TRCN0000004142 for human RNF12 knockdown. Immunofluorescence Cells were fixed for 10 min in 4% paraformaldehyde in PBS, permeabilized with 0.2% TritonX100-PBS and then blocked with 3% BSA in PBS for 30 min at room temperature. Specific first antibodies were diluted in 3% BSA-PBS and incubated with the slides for 3 h at room temperature (Flag, 1:500; NR4A1, 1:200; p-SMAD2 1:200, E-cadherin, 1:500). Secondary AlexaFluor488-labelled anti-mouse antibody (Molecular Probes) or AlexaFluor593-labelled anti-rabbit antibody (Molecular Probes) were added at a dilution of 1:200 in 3% BSA-PBS and incubated for 1 h at room temperature. Coverslips were mounted with VECTASHIELD mounting medium (Vector Laboratories Inc.). Fluorescence images were acquired with a Zeiss Axioplan microscope. The full western blots are shown in Supplementary Fig. 10 . Detection of membrane-associated TβRI Cells transfected or infected were biotinylated for 40 min at 4 °C and then incubated at 37 °C for various times. The biotinylated cell surface receptors were precipitated with streptavidin beads and analysed by anti-TβRI immunoblot. Ubiquitination assay Cells were washed with PBS and lysed in two pellet volumes of RIPA buffer (10 mM Na 2 HPO 4 , 10 mM NaH 2 PO 4 pH 7.4, 150 mM NaCl, 1% Triton, 0.5% sodium deoxycholate and 1% SDS) supplemented with protease inhibitors and 10 mM N -ethylmaleimide. Lysates were sonicated, boiled at 95 °C for 5 min, diluted with RIPA buffer containing 0.1% SDS and then centrifuged at 4 °C (16 × 10 3 g for 15 min). The supernatant was incubated with specific antibody and protein A-sepharose for 3 h at 4 °C. After extensive washing, bound proteins were eluted with 2 × SDS sample buffer and separated by SDS–polyacrylamide gel electrophoresis, followed by immunoblotting. Real-time quantitative RT–PCR Total RNAs were prepared using the NucleoSpin RNA II kit (BIOKÉ, the Netherlands). A total of 1 μg RNA was reverse-transcribed using the RevertAid First Strand cDNA Synthesis Kit (Fermentas). Real-time PCR was conducted with SYBR Green (Applied Bioscience) using a StepOne Plus real-time PCR system (Applied Bioscience). All of the values for target gene expression were normalized to GAPDH. The primers used in qRT–PCR were listed below: NR4A1 forward, 5′-AGGGCTGCAAGGGCTTCT-3′ NR4A1 reverse, 5′-GGCAGATGTACTTGGCGTTTTT-3′ AXIN2 forward, 5′-ATTCGGCCACTGTTCAGACG-3′ AXIN2 reverse, 5′-GACAACCAACTCACTGGCCTG-3′ GAPDH forward, 5′-CCATCCACAGTCTTCTGGGT-3′ GAPDH reverse, 5′-GATCATCAGCAATGCCTCCT-3′ mNR4A1 forward, 5′-TGCCCGTGGCTTTGGT-3′ mNR4A1 reverse, 5′-TGTGCAGGGACCGTGAGAA-3′ mSMAD7 forward, 5′-TGGATGGCGTGTGGGTTTA-3′ mSMAD7 reverse, 5′-TGGCGGACTTGATGAAGATG-3′ mAXIN2 forward, 5′-GGTTCCGGCTATGTCTTTGC-3′ mAXIN2 reverse, 5′-CAGTGCGTCGCTGGATAACTC-3′ mCTGF reverse, 5′-GGCCTCTTCTGCGATTTCG-3′ mCTGF forward, 5′-CCATCTTTGGCAGTGCACACT-3′ mGAPDH forward, 5′-AACTTTGGCATTGTGGAAGG-3′ mGAPDH reverse, 5′-ACACATTGGGGGTAGGAACA-3′. Chromatin immunoprecipitation assay ChIP assay was performed as described previously [9] , [43] . Cells grown to 100% confluence were crosslinked with 1% formaldehyde for 15 min at 37 °C; crosslinking reactions were quenched with 0.125 M glycine for 5 min at room temperature. Cells were rinsed twice with PBS and harvested with a silicon scraper. Cells were resuspended, lysed (1% SDS, 50 mM Tris–HCl; pH 8.0, 5 mM EDTA, protease inhibitors) and sonicated to obtain DNA fragments of ~300–500 bp long on average. Samples were then centrifuged at 14 × 10 3 r.p.m. for 10 min. The supernatant was diluted (20 mM Tris–HCl, pH 8.0, 2 mM EDTA, 1% Trion X-100, 150 mM NaCl and protease inhibitors) and pre-absorbed with 50 μl of protein A beads (Zymed). Supernatants were then incubated with 10 μg antibodies (as indicated) overnight at 4 °C. The immunocomplexes were collected with 100 μl of protein A beads in a 3-h co-incubation. Then, the mixture was washed sequentially with TSE I (0.1% SDS, 20 mM Tris–HCl pH 8.0, 2 mM EDTA, 1% Triton X-100, 150 mM NaCl and protease inhibitors), TSE II (0.1% SDS, 20 mM Tris–HCl pH 8.0, 2 mM EDTA, 1% Triton X-100, 500 mM NaCl and protease inhibitors), LiCl buffer (10 mM Tris–HCl pH 8.0, 1 mM EDTA, 0.25 mM LiCl, 0.1% NP-40 and 1% deoxycholate sodium) and TE (10 mM Tris–HCl pH 8.0, 1 mM EDTA pH 8.0). The bound immunocomplex was eluted by incubating with 400 μl of fresh elution buffer (25 mM Tris–HCl pH 8.0, 10 mM EDTA, 0.5% SDS) at 65 °C for 15 min with occasional vortexing. The crosslinking was reversed in an overnight incubation at 65 °C. Whole-cell extract (WCE) DNA (fraction reserved from the sonication step) was also subjected to crosslinking reversal. Immunoprecipitated DNA and WCE DNA were then purified by treating with RNaseA, proteinase K and multiple phenol:chloroform:isoamyl alcohol extractions. Immunoprecipitated DNA was analysed with absolute qRT–PCR and the amplification product was expressed as a percentage of the input (WCE) for each condition. The primers used to amplify the NR4A1-binding region of the hAXIN2 promoters were the following: hAXIN2 promoter, forward 5′-TGAAGTCCCAGCTGGTGTGA-3′ and reverse 5′-TGACCTTTAGTCAGCCCCACAAA-3′; mAXIN2 promoter, forward 5′-GCAGCTGTGGAACCTTTTATGA-3′ and reverse 5′-GCTAAGATCCAAGACGAAGTTTGAC-3′. Primers used for the control region were the following: forward 5′-TTGAGATGGAGTCTTGCTCTG-3′ reverse: 5′-GTGAAACCCTGTCCCTACTAAA-3′. Migration and invasion assays Transwell assay was performed in 24-well PET inserts (Falcon 8.0 μm pore size) for migration assay. MDA-MB-231 stable cells were serum starved overnight. Then, 50 × 10 3 or 10 × 10 3 cells were plated in transwell inserts (at least three replicas for each sample) and left treated with or without SB431542 (5 μM) for 8 h. Cells in the upper part of the transwells were removed with a cotton swab; migrated cells were fixed in paraformaldehyde 4% and stained with crystal violet 0.5%. Filters were photographed and the total number of cells was counted. Every experiment was repeated at least three times independently. Zebrafish embryonic invasion and metastasis assay We used a zebrafish embryo xenograft model developed by Snaar–Jagalska and collegues [44] , where mammalian tumour cells are injected into the zebrafish embryonic blood circulation. Animal Experiments Committee (DEC) of the LUMC approved the studies using Zebrafish (Danio rerio ). The zebrafish were handled and maintained in compliance with the local animal welfare regulations and to standard protocols. Experiments were performed as described previously [31] . mCherry stably expressed-MDA-MB-231 cells were infected with control or NR4A1 shRNA lentivirus for 2 days and then puromycin selected for another 3 days. The in vitro proliferation rate of shRNA NR4A1 cells was similar to that of control cells. Before injection, cells were treated with IL-1β (10 ng ml −1 ) or TNF-α (10 ng ml −1 ) for 6 h. IL-1β− and TNF-α-treated cells did not show significant differences in in vitro proliferation as compared with control cells. Approximately 400 tumour cells were injected into the blood of 48 h post fertilization Fli-Casper zebrafish embryos at the ducts of Cuvier. After injection, some of the tumour cells disseminate into the embryo blood circulation while the rest remain in the yolk. Zebrafish embryos are maintained for 5 days post injection at 33 °C, a compromise for both the fish and cell lines. The tumour cells that enter into the blood stream preferentially invade and micrometastasize into the posterior tail fin area. Invasion can be visualized as a single cell that has left the blood vessel, which can subsequently form a micrometastasis (3~50 cells). Pictures were taken by confocal microscopy at 1, 3 and 5 days post injection and the percentage of invasion and micrometastasis were counted. Every experiment was repeated at least two times independently. Mice metastasis model MDA-MB-231 cells were infected with control or NR4A1 shRNA lentivirus for 2 days and puromycin was selected for another 3 days. Cells were pretreated with IL-1β (10 ng ml −1 ) for 6 h before injection. A single-cell suspension of MDA-MB-231/luc cells (1 × 10 5 per 100 μl PBS) was inoculated into the left heart ventricle ( n =10) according to the method described by Arguello et al. [45] Cells were injected into female mice at the age of 5 weeks. Animals in which cardiovascular injection/misinjection caused immediate death were excluded from further analysis (usually 6< n <10). Development of metastases was monitored weekly by bioluminescent reporter imaging. After 6 weeks, all mice were killed and metastases were dissected. Animal experiments were approved by the Institutional Committee for Animal Welfare of the LUMC and were performed according to the regulatory guidelines. Statistical analysis Student’s t -tests were performed for statistical analyses. Data in all graphs are presented as means±s.d. Pearson’s coefficient tests were used to analyse correlation between NR4A1 and related genes. Analysis of variance was used to analyse zebrafish experiments. Spearman’s correlation test was used to analyse the relationships between NR4A1 and p-SMAD2. How to cite this article: Zhou, F. et al. Nuclear receptor NR4A1 promotes breast cancer invasion and metastasis by activating TGF-β signalling. Nat. Commun. 5:3388 doi: 10.1038/ncomms4388 (2014).